Re-engineered BCG overexpressing cyclic di-AMP augments trained immunity and exhibits improved efficacy against bladder cancer 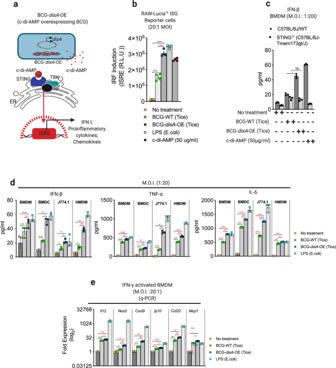Fig. 1: BCG-disA-OE elicits greater pro-inflammatory cytokine responses than BCG-WT in primary human and murine macrophages and dendritic cells in vitro. aSchematic diagram.bIRF3 induction measured in RAW-Lucia ISG reporter macrophages.cIFN-β levels in murine BMDM from wild-type and STING−/−mice.dIFN-β, TNF-α, and IL-6 levels from primary human and murine macrophages and dendritic cells and the J774.1 murine macrophage cell line.emRNA levels for Th1 cytokines and chemokines in murine BMDM relative to β-actin. Cytokine levels were measured by ELISA after 24 h exposures at a MOI of 20:1. Transcript levels were measured at 6 h after infection. Data are presented as mean values ± S.E.M. (n= 3 biological replicate experiments). Statistical analyses done using two-tailed Student’st-test (*P< 0.05, **P< 0.01, ***P< 0.001, ****P< 0.0001). Data shown are for BCG-Tice; similar findings were observed for BCG-Pasteur as shown in Fig. S2. In addition to its role as a TB vaccine, BCG has been shown to elicit heterologous protection against many other pathogens including viruses through a process termed trained immunity. Despite its potential as a broadly protective vaccine, little has been done to determine if BCG-mediated trained immunity levels can be optimized. Here we re-engineer BCG to express high levels of c-di-AMP, a PAMP recognized by stimulator of interferon genes (STING). We find that BCG overexpressing c-di-AMP elicits more potent signatures of trained immunity including higher pro-inflammatory cytokine responses, greater myeloid cell reprogramming toward inflammatory and activated states, and enhances epigenetic and metabolomic changes. In a model of bladder cancer, we also show that re-engineered BCG induces trained immunity and improved functionality. These results indicate that trained immunity levels and antitumor efficacy may be increased by modifying BCG to express higher levels of key PAMP molecules. Although it was developed in 1921 as a tuberculosis vaccine, BCG has been found to elicit non-specific protection against a host of heterologous infections, including viral infections. In both prospective and retrospective human studies, BCG has been shown to reduce rates of RSV, HSV, HPV, and other viruses [1] . A recent prospective study of BCG administration to elderly patients showed a statistically significant reduction in all-cause infections compared with placebo [2] . Indeed, there is a growing body of evidence that BCG may protect against COVID-19 [3] , [4] , [5] , and a number of prospective clinical trials of BCG for COVID-19 prevention are currently ongoing [6] . BCG has also been used as a cancer therapeutic for solid organ malignancies due to this heterologous protection [7] . This phenomenon of BCG-mediated, heterologous protection has been termed “trained immunity” [8] since it can be demonstrated that following BCG uptake myeloid cells are reprogrammed or trained to an altered immune setpoint to respond to subsequent pathogen challenges. BCG-mediated training also occurs in myeloid precursors in the bone-marrow suggesting a basis for the durable protection observed [9] , [10] . Among the hallmarks of trained immunity are elevated levels of pro-inflammatory cytokine release, macrophage reprogramming towards inflammatory, activated phenotypes, epigenetic changes, which are pro-inflammatory, and metabolomic changes towards enhanced glycolysis [11] . The ability to elicit trained immunity is not restricted to BCG, and the phenomenon has been observed with viral vaccines such as the live oral polio vaccine, Candida albicans infections, and also a number of PAMPs, including zymosan, β-glucan, and LPS [12] . While precise mechanisms for how BCG and other trained immunity-stimulating microbes elicit epigenetic and metabolomic reprogramming, it has been shown that pattern recognition receptor (PRR) engagement of molecules such as dectin-1 and TLR4 is an early event [13] . Recently, the transcription factor C/EBPβ was demonstrated to mediate chromatin accessibility memory in the training of hematopoietic stem cells by LPS and TLR4, thus providing a mechanistic link between PRR engagement and epigenetic modifications [14] . Despite the potential for BCG and other trained immunity agents to serve as broadly protective vaccines and immunoadjuvants, little has been done to determine if BCG-mediated trained immunity levels may be enhanced. In this study, we sought to determine if a re-engineered BCG might offer enhanced trained immunity. To address this question, we generated a recombinant BCG that releases high levels of cyclic-di-AMP (c-di-AMP), a PAMP that is recognized by the PRR, stimulator of interferon genes (STING). We compared the recombinant BCG overexpressing cyclic-di-AMP (hereafter abbreviated BCG- disA -OE) with an otherwise isogenic wild-type BCG (BCG-WT). Our results show that engineering BCG to express high levels of cyclic-di-AMP dramatically increases trained immunity levels scored across multiple parameters with human and murine primary cells. The cyclic-di-AMP overexpressing strain was also more potent in vivo as an immunotherapy in models of urothelial cancer where BCG is clinically used. While BCG- disA -OE has previously been shown to elicit enhanced protection against tuberculosis disease progression compared to BCG-WT in the guinea pig model [15] and a related BCG in the mouse model [16] , its ability to elicit trained immunity responses and to act as a bladder cancer immunotherapy has not been previously evaluated. BCG- disA -OE elicits greater pro-inflammatory cytokine responses in macrophages than BCG-WT BCG- disA -OE is a genetically engineered BCG strain in which an endogenous diadenylate cyclase gene, disA , is fused to a strong promoter, leading to a 300-fold overexpression of disA and a 15-fold increase in production of cyclic-di-AMP (Fig. 1a and Fig. S1a ) [17] . Compared with BCG-WT, BCG- disA -OE significantly increased STING pathway activation in macrophages as measured by IRF3 induction (Fig. S1b ). To control for the fact that numerous BCG strains are used worldwide and variabilities in their clinical efficacies have been described, we generated two versions of BCG- disA -OE and a corresponding BCG-WT: one using BCG-Tice (data shown in the main figures) and one using BCG-Pasteur (data shown in the supplementary figures). We did not detect significant differences between the Tice and Pasteur versions. Fig. 1: BCG- disA -OE elicits greater pro-inflammatory cytokine responses than BCG-WT in primary human and murine macrophages and dendritic cells in vitro. a Schematic diagram. b IRF3 induction measured in RAW-Lucia ISG reporter macrophages. c IFN-β levels in murine BMDM from wild-type and STING −/− mice. d IFN-β, TNF-α, and IL-6 levels from primary human and murine macrophages and dendritic cells and the J774.1 murine macrophage cell line. e mRNA levels for Th1 cytokines and chemokines in murine BMDM relative to β-actin. Cytokine levels were measured by ELISA after 24 h exposures at a MOI of 20:1. Transcript levels were measured at 6 h after infection. Data are presented as mean values ± S.E.M. ( n = 3 biological replicate experiments). Statistical analyses done using two-tailed Student’s t -test (* P < 0.05, ** P < 0.01, *** P < 0.001, **** P < 0.0001). Data shown are for BCG-Tice; similar findings were observed for BCG-Pasteur as shown in Fig. S2. Full size image To characterize the trained immunity-inducing potential of BCG- disA -OE versus BCG-WT, we evaluated their capacity to induce cytokine expression in human monocyte-derived macrophages (HMDMs), primary murine bone-marrow-derived macrophages (BMDM), and dendritic cells (BMDC) as well as a macrophage cell line (J774.1). We found consistent induction of IRF3, IFN-β, TNF-α, and IL-6 in all myeloid cell types in response to BCG- disA -OE that was significantly higher than that seen with BCG-WT-exposed cells (Fig. 1b–d and Fig. S2a, b ), and in human MDM and murine BMDM this difference was observed even in when cells were IFN-γ primed (Fig. S2c, d ). These differences were strictly STING-dependent as confirmed using BMDM from STING −/− mice (Fig. 1c ). Since STING activation leads to upregulation of NF-κB via the TBK1-IRF3 pathway, we found that expression of both TNF-α and IL-6 in the same panel of cells paralleled that of IFN-β and was significantly higher following exposure to BCG- disA -OE compared with BCG-WT (Fig. 1d and S2b ). Cyclic dinucleotides including cyclic-di-AMP are known to be potent inducers of several chemokines (CXCL9, CXCL10 [IP-10], CXCL22, and MCP-1) as well as iNOS [18] , [19] ; consistent with this, IFN-γ-primed BMDMs showed a more robust induction of these chemokines and Nos2 when challenged with BCG- disA -OE strain than with BCG-WT (Fig. 1e ). We also assessed the cellular toxicity using annexin-PI staining and found that whereas late apoptotic cell death remained at baseline with BCG- disA -OE exposure in both BMDM and J774.1 macrophages, BCG-WT exposure elicited significantly higher levels of apoptotic cell death (Fig. S3a, b ) in the BMDM cells. These observations demonstrate that BCG- disA -OE elicits pro-inflammatory cytokine expression more potently than BCG-WT in primary human MDM, as well as murine primary macrophages and macrophage cell lines. Pro-inflammatory polarization of macrophages is greater with BCG- disA -OE than with BCG-WT Trained immunity is associated with polarization of macrophages towards inflammatory phenotypes with a concomitant shift away from anti-inflammatory states [12] . To investigate macrophage polarization, we used flow-cytometry to monitor phenotypic shifts of both murine and human primary macrophages following a 24 h exposure to BCG- disA -OE or BCG-WT. First, we focused on the MHC class-II-expressing CD45 + CD11b + F4/80 + murine BMDM population following in vitro BCG exposure using the gating scheme shown in Fig. S4a, b . As may be seen in Fig. 2a and Fig. S5a, b , we observed a significantly greater expansion of TNF-α-expressing CD11b + F4/80 + inflammatory murine BMDMs following exposure to BCG- disA -OE than with BCG-WT. We next gated on cells expressing the immunosuppressive surface receptors CD206 + and CD124 + among CD45 + CD11b + F4/80 + macrophages and observed a greater reduction of this population with BCG- disA -OE than with to BCG-WT (Fig. 2a and Fig. S5c, d ). Within this immunosuppressive cell population, there was a higher proportion of IL-10-expressing CD206 + CD124 + cells in BCG-WT-exposed macrophages, while IL-10-expressing cells were significantly reduced in response to BCG- disA -OE exposure (Fig. 2a and Fig. S5e, f ). These results demonstrate that compared with BCG-WT, BCG- disA -OE exposure elicits more extensive macrophage reprogramming with expansion of pro-inflammatory macrophages displaying increased antigen presentation (MHC class-II expression) and TNF-α expression and contraction of immunosuppressive macrophages expressing IL-10. Fig. 2: BCG- disA -OE elicits greater macrophage reprogramming, phagocytic activity, and autophagy than BCG-WT in human and murine macrophages. a Percentages of inflammatory M1- and immunosuppressive M2-macrophages and M-MDSCs arising from primary murine macrophages. b Percentages of inflammatory, TNF-α + M1, and IL-6 + inflammatory macrophages (M1-like), and c CD206 + CD124 + and IL-10 + immunosuppressive macrophages (M2-like) arising from primary human macrophages. Data were collected after 24 h exposures at MOI of 20:1 as determined by flow-cytometry using gating schemes shown in Fig. S3 – S9 . Data are presented as mean values ± S.E.M. ( n = 4 independent biological replicate experiments). d Phagocytic activity in human primary macrophages in representative confocal photomicrographs showing intracellular uptake of FITC-labeled IgG-opsonized latex beads (green) with nuclei stained blue. Data are represented as mean values ± S.E.M ( n = 3 independent biological replicate experiments). e Autophagy induction and f quantification by BCG-LC3B colocalization in primary murine macrophages shown by representative confocal photomicrographs. Autophagy was measured by LC3B puncta or g . p62 colocalization with BCG appearing in yellow. FITC-labeled BCG strains are stained green, LC3B or p62 autophagic puncta (red), and nuclei blue. h Quantification of BCG-p62 colocalization. Cells were fixed using 4% paraformaldehyde 6 h after infection (MOI 10:1), and images obtained with an LSM700 confocal microscope and Fiji software processing. Quantification was measured by mean fluorescence intensity. Data represented for all confocal microscopy studies (phagocytosis, LC3B-BCG colocalization and p62-BCG colocalization) as mean values ± S.E.M. ( n = 3 independent biological replicate experiments). All statistical analyses done using two-tailed Student’s t -test (* P < 0.05, ** P < 0.01, *** P < 0.001, **** P < 0.0001). Data shown are for BCG-Tice; similar findings were observed for BCG-Pasteur as shown in Figs. S2 and S7 . Full size image Myeloid-derived suppressor cells (MDSCs) are a heterogeneous population of immature myeloid cells known to foster immunosuppression [20] , [21] . Accordingly, we investigated the induction of monocytic-myeloid-derived suppressor cells, M-MDSCs, (CD45 + Ly6C hi Ly6G - CD11b + F4/80 - ) using primary murine BMDMs using the gating scheme shown in Fig. S6 . Following BCG-WT exposure we observed a significant expansion of M-MDSCs, while in contrast this same population showed minimal expansion following BCG- disA -OE exposure (Fig. 2a and Fig. S7a, b ). Moreover, the M-MDSCs elicited by BCG-WT exhibited higher IL-10 expression, whereas IL-10-expressing M-MDSCs were virtually absent after BCG- disA -OE exposure (Fig. 2a and Fig. S7c, d ). These observations suggest that BCG-WT contributes to an expansion of M-MDSCs, which have immunosuppressive properties; however, forced overexpression of the pro-inflammatory PAMP cyclic-di-AMP by BCG prevents M-MDSC expansion. We next characterized the macrophage activation phenotypes in HMDMs isolated from several independent healthy human donors. Both the BCG-WT and BCG- disA -OE strains elicited increases in the population of classical macrophages (CD11b + CD14 + CD16 − ), but these inductions were comparatively higher in response to BCG- disA -OE (Fig. 2b and Fig. S8a–c ). We examined classically activated antigen-presenting macrophages (CD14 + CD16 − HLA-DR + ) and their ability to produce TNF-α or IL-6 and found a significantly increased proportion of TNF-α and IL6- producing HLA-DR + cells following exposure to BCG- disA -OE compared to BCG-WT (Fig. 2b and Fig. S9a, b ). We also investigated the immunosuppressive surface markers, CD206 + and CD163 + , on transitional or intermediate macrophages (CD11b + CD14 + CD16 + ) and found a consistently greater decrease in them following BCG- disA -OE exposure than with BCG-WT (Fig. 2c ; Figs. S8b and S9b ). The fraction of these intermediate macrophages expressing immmunosuppressive surface markers and IL-10 was also significantly lower in response to exposure to BCG- disA -OE than with BCG-WT (Fig. 2c and Fig. S9b ). In summary, using both mouse and human primary macrophage ex vivo models, we found that, compared with BCG-WT, BCG- disA -OE promotes greater macrophage activation towards an inflammatory phenotype, and concomitantly reduces the emergence of cells with immunosuppressive abilities, including M-MDSCs. Macrophages exposed to BCG- disA -OE are more phagocytic than those with BCG-WT Cyclic dinucleotides have been reported to recruit inflammatory macrophages that display high phagocytic potential [22] , [23] , [24] , [25] . Consistent with these observations we confirmed that HMDMs transfected with cyclic-di-AMP showed increased phagocytosis and exhibited elongated dendrites compared to mock-transfected populations (Fig. S10 ). We then evaluated the phagocytic properties of HMDMs following exposure to the different BCG strains and found significantly greater phagocytosis of IgG-opsonized FITC-latex beads by macrophages exposed to BCG- disA- OE compared to BCG-WT (Fig. 2d ). In keeping with the previously established role of STING pathway activation in augmenting autophagy [17] , [26] , [27] , we found that a majority of intracellular BCG- disA -OE bacilli were co-localized with LC3B in IFN-γ-activated primary BMDMs (Fig. 2e, f ), while autophagy induction in BCG-WT was significantly lower. We also found significantly greater colocalization of BCG- disA -OE bacilli with the autophagy adapter protein p62 compared to that observed with BCG-WT (Fig. 2g, h ). These results reveal BCG- disA -OE increases the levels of phagocytosis and autophagic processing within macrophages to a greater degree than BCG-WT, a phenomenon associated with enhanced peptide antigen presentation to MHC class-II molecules [28] , [29] . BCG- disA -OE reprograms macrophages epigenetically and potentiates trained immunity to a greater degree than BCG-WT In light of recent data showing BCG to be a potent inducer of trained immunity through epigenetic modifications of key pro-inflammatory genes [9] , [30] , [31] we hypothesized that the addition of cyclic-di-AMP overexpression to standard BCG might potentiate epigenetic modifications in primary human monocytes. Having already established that BCG- disA -OE is a more potent inducer of macrophage TNF-α and IL-6 secretion than BCG-WT, we confirmed this in primary human monocytes from a group of 6 healthy human subjects (Fig. 3a ). The ability of traditional BCG to elicit trained immunity has been correlated with changes in epigenetic marks that increase pro-inflammatory gene expression [32] . Thus, we asked if the enhanced induction of TNF-α and IL-6 expression elicited by BCG- disA -OE compared with BCG-WT is epigenetically mediated. To this end, we evaluated the promoter regions of the TNF-α and IL-6 genes for durable, antigen-independent epigenetic changes using an assay [33] in which human monocytes exposed to BCG strains for 24 h were rested for five days prior to challenge with a heterologous antigen, the TLR1/2 agonist Pam3CSK4 on day 6 (Fig. 3b ). Using chromatin immunoprecipitation-polymerase chain reaction (ChIP-PCR) assays, we quantified the activating histone methylation mark H3K4me3 present in the TNF-α and IL-6 promoters. We observed that exposure to BCG- disA -OE led to greater enrichment of this mark than BCG-WT even without the heterologous second stimulation (i.e., adding RPMI media alone at day 6). Upon re-stimulation with Pam3CSK4 at day 6, the abundance of the activating epigenetic mark was further increased by both BCG strains, but BCG- disA -OE-pretreatment yielded notably more enrichment than BCG-WT (Fig. 3c ). Similarly, we investigated the chromatin repression mark H3K9me3 at the same two promoters and found that, while both BCG strains led to reduced levels of H3K9me3 (which were further accentuated by addition of Pam3CSK4), the degree of reduction mediated by BCG- disA -OE was consistently greater than that mediated by BCG-WT, both upon initial exposure and after rest and re-stimulation (Fig. 3d ). Simultaneous measurement of TNF-α and IL-6 in BCG-trained culture supernatant following non-specific stimulation by Pam3CSK4 revealed that BCG- disA -OE-trained macrophages produced significantly higher levels of these pro-inflammatory cytokines than did those trained with BCG-WT (Fig. 3e, f ). These results indicate that an augmented BCG that overexpresses the PAMP molecule cyclic-di-AMP leads to significantly more robust epigenetic changes classically associated with trained immunity. Fig. 3: Compared with BCG-WT, BCG- disA -OE is a more potent inducer of epigenetic changes characteristic of trained immunity in primary human monocytes. a mRNA levels of TNF-α and IL-6 in primary human monocytes ( n = 6 healthy donors) relative to RNU6A after 24 h exposures at a MOI of 10:1. Statistical analysis done using multiple unpaired t-test with Bonferroni-Dunn method. b Schematic diagram of in vitro monocyte training. c Relative levels of the H3K4me3 chromatin activation mark ( n = 4 healthy donors; D1–D4) or d the H3K9me3 chromatin repression mark retrieved from TNF-α and IL-6 promoter regions of primary human monocytes from 3 ( n = 3) health donors (D1–D3) determined by ChIP-PCR assay on day 6. e , f Secreted cytokines (TNF-α and IL-6) following BCG training and re-stimulation. Monocytes were initially challenged on day 0 with a 24 h exposure to the BCG strains at a MOI of 10:1 followed by washing. After 5 days of rest, they were treated for 24 h with either a sham stimulus (RPMI) or the TLR1/2 agonist Pam3CSK4 ( n = 3 healthy donors). Data are presented as mean values ± S.E.M. Statistical analyses done using two-tailed Student’s t -test (* P < 0.05, ** P < 0.01, *** P < 0.001, **** P < 0.0001). Full size image BCG- disA -OE reprograms the macrophage immuno-metabolic state towards pro-inflammatory signatures to a greater degree than BCG-WT BCG-training has been reported to stimulate glycolysis as well as the tricarboxylic acid cycle through glutamine replenishment with accumulation of fumarate [34] . To address whether the addition of cyclic-di-AMP overexpression alters the BCG-mediated metabolomic shifts, we used LC-MS to characterize key metabolites in primary human and murine macrophages exposed to the two BCG strains. As shown in Fig. 4a, b , HMDMs or BMDMs showed increased catabolic signatures (elevated intracellular glucose and lactate) to a greater degree following a 24 h exposure to BCG- disA -OE than with BCG-WT. Also, the TCA cycle metabolites itaconate and fumarate were also more elevated with BCG- disA -OE than with BCG-WT (Fig. 4c ). These observations suggest greater catabolism of carbon substrates for ATP generation consistent with a pro-inflammatory bioenergetic profile in macrophages infected with BCG- disA -OE than with BCG-WT [35] . Fig. 4: Compared with BCG-WT, BCG- disA -OE is a more potent inducer of metabolomic changes characteristic of trained immunity in primary human monocytes. a , b Metabolite levels determined by LC-MS in human ( n = 2 independent biological replicate), or murine MDM ( n = 4 independent biological replicate experiments) determined 24 h after exposure to BCG strains or heat-killed controls. The data are presented as mean values ± S.E.M. Cartoon diagram c showing key metabolites significantly upregulated (red arrow upward) or downregulated (blue arrow downward) in BCG- disA -OE infected macrophages relative to BCG-WT infected macrophages. Statistical analyses done using two-tailed Student’s t- test (* P < 0.05). Full size image In order to determine whether the elevated levels of intracellular glucose were due to increased transport or to increased gluconeogenesis, we tested expression of the major glucose transporter GLUT1 in macrophages exposed to BCG-WT and BCG- disA -OE. As shown in Fig. S11a , we challenged murine BMDM with BCG or BCG- disA -OE for 4 h, and after washing and recovery in glucose-free media, macrophages were treated with the fluorescent 2-deoxy-glucose analog 2-NBDG for 2 h and subsequently analyzed by flow-cytometry for levels of GLUT1 expression or 2-NBDG uptake. As may be seen in Fig. S11b , exposure to BCG-WT and BCG- disA -OE led to a 2-fold and more than a 5-fold increase, respectively, of GLUT1 expression on BMDM compared to unexposed cells. Similarly, 2-NBDG levels were elevated by 20% or 40% following exposure to BCG-WT and BCG- disA -OE, respectively as shown in Fig. S11c . These observations strongly suggest that BCG- disA -OE elicits higher levels of the GLUT1 transporter and glucose uptake than BCG-WT or untreated controls resulting in greater accumulation of intracellular glucose and are consistent with earlier observations linking trained immunity and STING activation with enhanced mTOR-HIF-1α pathway activation and concomitant elevations in glucose transporter levels [32] , [36] , [37] . Excess tryptophan catabolism to kynurenine by tryptophan dehydrogenase and indoleamine 2,3-dioxygenase (IDO) has been strongly associated with immunosuppression [38] , and IDO inhibitors have shown potential as immune activators in a variety of infectious and oncologic diseases [39] . Kynurenine levels were dramatically lower in macrophages following BCG- disA -OE exposure than those seen with BCG-WT (Fig. 4a ), and as would be expected tryptophan levels were elevated by BCG- disA -OE while BCG-WT led to tryptophan levels comparable to the baseline seen with heat-killed BCG controls (Fig. 4b ). Citrulline levels were also higher while putrescine levels were lower with BCG- disA -OE than BCG-WT, suggesting that nitric oxide synthase-mediated conversion of arginine to NO (pro-inflammatory) and citrulline was more strongly induced by BCG- disA -OE (Fig. 4c ). Finally, it was of interest that itaconate, an isocitrate lyase inhibitor made by macrophages that has been shown to have antibacterial activity, was more potently induced by BCG- disA -OE than BCG-WT (Fig. 4c ). Thus, compared with BCG-WT, BCG- disA -OE elicited a greater pro-inflammatory metabolomic signature with reduced kynurenine accumulation and increases in glycolytic metabolites, NOS products, and itaconate production. Functional efficacy in vivo: BCG- disA -OE demonstrates superior immunotherapeutic outcomes in relevant animal models of trained immunity In addition to being used as a TB vaccine, BCG has served as a first-line immunotherapy for the treatment of non-muscle invasive bladder cancer (NMIBC) since the mid-1970s. Recent studies have indicated that BCG exerts its antitumor effects via a trained immunity mechanism [40] . Having demonstrated that augmenting BCG with excess cyclic-di-AMP release leads to improved trained immunity parameters across a battery of in vitro assays, we sought to determine if these effects could be demonstrated in vivo. First, we tested BCG- disA -OE versus BCG-WT in a carcinogen-induced model of NMIBC in which intravesical therapies can be introduced into the bladder as they are in humans with non-invasive urothelial cancer. The rat N -methyl- N -nitrosourea (MNU) model of bladder cancer (BC) is schematized in Fig. 5a [41] , [42] , [43] In this model urothelial dysplasia develops at week 14 after the first intravesical instillation of MNU and by week 24 rats display a different forms of urothelial cancer severity including carcinoma-in-situ (CIS), papillary Ta (superficial), or higher-grade T1-T2 urothelial carcinoma with histopathologic and immunophenotypic features similar to those observed in human bladder cancer [41] , [42] , [44] . Following carcinogen-mediated tumor induction with 4 weekly cycles of MNU (wk 0, wk 2, wk 4, wk6), groups of rats were treated with 6 weekly doses of intravesical BCG- disA -OE, BCG-WT, or no treatment from week 18–23. Upon sacrifice at wk 24 we divided the rat urinary bladders into halves for (i) reverse transcription–polymerase chain reaction (RT-PCR) analysis, and (ii) histologic analysis including tumor staging by a blinded genitourinary pathologist. Transcriptional analysis of the whole excised bladders at week 24 showed that compared with BCG-WT, BCG- disA -OE elicited significantly increased levels of Ifnb , Ifng , Tnfa , Il1b , Cxcl10 , Mcp1 , Mip1a and Nos2 transcription while mRNA levels of the immunosuppressive cytokines Il10 and Tgfb were reduced by both BCG strains (Fig. 5b ) We confirmed these patterns of cytokine expression at the protein level using enzyme-linked immunosorbent assay (ELISA) for TNF-α, IL-2, and IFN-γ, and noted that intravesical BCG- disA -OE, strongly increased the levels of IFN-γ in rat spleens while BCG-WT did not (Fig. S12a ). Correspondingly, we found a significant decrease in highest pathology grade (Fig. 5c ), tumor involvement index (Fig. 5d ) and highest tumor stage (Fig. 5e ) in MNU rats treated with BCG- disA -OE in comparison to untreated. By tumor involvement index BCG- disA -OE was statistically significantly superior to no treatment ( P < 0.001) and to BCG-WT ( P < 0.05), whereas BCG-WT showed only a trend towards improvement over no treatment. Importantly, the highest tumor stage observed in BCG- disA -OE-treated rats was CIS, whereas it was T1 in those receiving BCG-WT, and T2 in untreated rats, and 53.3% of BCG- disA -OE-treated rats were cancer free ( P = 0.009) compared with 31.2% of BCG-WT and 0% of the untreated rats (Fig. 5e ). Immunohistochemical analyses revealed a significant reduction in Ki67 staining in BCG- disA -OE-treated MNU rat bladders when compared to untreated ( P < 0.01) and BCG-WT ( P < 0.05), suggesting reduced tumor proliferation (Fig. 5f ). CD68 staining of rat bladder showed significantly higher levels of macrophage recruitment with a trend toward elevation of the pro-inflammatory CD86 + macrophages (Fig. 5g ) and a significant reduction in CD206 + immunosuppressive (M2-like) macrophages that are associated with tumor promotion in the BCG- disA -OE-treated rats compared with untreated controls. These observations indicate that the enhanced induction of type I IFN and other pro-inflammatory signatures in bladders of tumor-bearing rats treated with BCG- disA -OE correlated with the enhanced antitumor activity of the recombinant BCG strain. Fig. 5: BCG- disA -OE elicits improved antitumor efficacy over BCG-WT in the orthotopic carcinogen-induced rat model of urothelial cancer. a Schematic diagram of the MNU rat model of NMIBC. b mRNA levels for pro-inflammatory cytokines ( Ifnb , Ifng , Tnfa , and Il1b ), regulatory chemokines ( Cxcl10 , Mcp1 , and Mip1a ), immunosuppressive M2-like macrophage cytokines ( Il10 and Tgfb ) and M1-like tumoricidal effectors ( Nos2 ) in whole bladders at necropsy (wk 23) measured by qRT-PCR relative to GAPDH ( n = 5 animals/group). c Representative H&E staining showing highest pathology grade for each group [control, untreated MNU bladder, BCG-WT (Past and Tice), and BCG- disA -OE (Past and Tice) ( n = 12–16 animals/group)]. d Tumor involvement values at necropsy (7–11 animals/group). e Highest tumor stage at necropsy. f Representative immunohistochemistry and bar graph of rat bladder tissue at necropsy stained for Ki67 ( n = 17–22 animals). g Representative immunohistochemical co-staining and line graph for CD68 (brown), CD86 (M1-like macrophages; red) and CD206 (M2-like macrophages; red) in rat bladder tissues at necropsy ( n = 5 animals per group). Data are presented as mean values ± S.E.M. (qRT-PCR) or mean values ± S.D. (tumor involvement index, Ki67 staining and IHC scores). Statistical analyses done using two-tailed Student’s t- test (* P < 0.05, ** P < 0.01, *** P < 0.001, **** P < 0.0001) (qRT-PCR) and one-way ANOVA (## P < 0.01). Full size image We also tested the functional efficacy of BCG- disA -OE in a murine heterotopic, syngeneic urothelial cancer model using MB49 urothelial cancer cells. Following flank engraftment with MB49 tumor cells, mice received four intratumoral treatments over 9 days as shown in Fig. 6a . In this model BCG- disA -OE also showed more robust immunotherapeutic efficacy than BCG-WT as measured by tumor volume and weight after intratumoral injection of BCG- disA -OE when compared with BCG-WT (Fig. 6b and Fig. S13a ). Histopathology demonstrated extensive necrosis and congestion in MB49 tumors treated with BCG- disA -OE when compared to BCG-WT and untreated (Fig. S13b ). There were no significant changes in body weights of mice receiving BCG, however splenic weight was significantly increased by both BCG strains (Fig. S13c ). We further characterized the impact of the treatments on macrophage polarization and recruitment of activated T cells in the tumor microenvironment (TME). As shown in Fig. 6c , compared with BCG-WT, BCG- disA -OE significantly reduced the abundance of immunosuppressive macrophages (CD206 + CD124 + ) when compared to untreated and BCG-WT and significantly ( P < 0.01) increased pro-inflammatory macrophages (TNF-α + MHCII + ). Similarly, BCG- disA -OE recruited significantly more IFN-γ-producing CD4 + T cells when compared to BCG-WT, and both BCG strains increased IFN-γ-producing CD8 + T cells. While both BCG strains recruited more CD4 + and CD8 + cells to the tumors, BCG- disA -OE uniquely recruited more CD8 + T cells to the spleens of treated animals (Fig. S13d ). BCG- disA -OE also significantly reduced tumor-associated T-regulatory (Treg) cells to a greater degree than BCG-WT in both tumor and spleen (Fig. S13e ). In keeping with our earlier findings in primary cells, we also found that compared with BCG-WT, BCG- disA -OE elicited more potent cytokine responses and autophagy in human urothelial cancer cells representing various tumor stages (Fig. S14a–e ). These results indicate that in this murine model of urothelial cancer, BCG- disA -OE has superior antitumor efficacy than BCG-WT, and its efficacy correlates with shift in polarization of macrophages to more inflammatory states, increased activation of both CD4 + and CD8 + T cells, and a reduction of local intratumoral and systemic Treg cell populations. Fig. 6: BCG- disA -OE elicits improved antitumor efficacy over BCG-WT in the syngeneic MB49 heterotopic mouse model of urothelial cancer. a Schematic diagram of the syngeneic MB49 mouse model of urothelial cancer. b MB49 tumor volume and tumor weight at time of necropsy ( n = 9 animals per group). c Tumor-infiltrating M1 and M2 macrophages and CD4 and CD8 T-cell lymphocyte types at necropsy in the MB49 model ( n = 9 animals per group). Data are presented as mean values ± S.E.M. Statistical analyses for tumor volume data were done using one-way ANOVA (* P < 0.05, ** P < 0.01, *** P < 0.001, **** P < 0.0001). 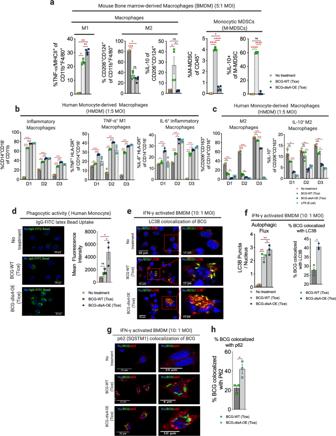Fig. 2: BCG-disA-OE elicits greater macrophage reprogramming, phagocytic activity, and autophagy than BCG-WT in human and murine macrophages. aPercentages of inflammatory M1- and immunosuppressive M2-macrophages and M-MDSCs arising from primary murine macrophages.bPercentages of inflammatory, TNF-α+M1, and IL-6+inflammatory macrophages (M1-like), andcCD206+CD124+and IL-10+immunosuppressive macrophages (M2-like) arising from primary human macrophages. Data were collected after 24 h exposures at MOI of 20:1 as determined by flow-cytometry using gating schemes shown in Fig.S3–S9. Data are presented as mean values ± S.E.M. (n= 4 independent biological replicate experiments).dPhagocytic activity in human primary macrophages in representative confocal photomicrographs showing intracellular uptake of FITC-labeled IgG-opsonized latex beads (green) with nuclei stained blue. Data are represented as mean values ± S.E.M (n= 3 independent biological replicate experiments).eAutophagy induction andfquantification by BCG-LC3B colocalization in primary murine macrophages shown by representative confocal photomicrographs. Autophagy was measured by LC3B puncta org. p62 colocalization with BCG appearing in yellow. FITC-labeled BCG strains are stained green, LC3B or p62 autophagic puncta (red), and nuclei blue.hQuantification of BCG-p62 colocalization. Cells were fixed using 4% paraformaldehyde 6 h after infection (MOI 10:1), and images obtained with an LSM700 confocal microscope and Fiji software processing. Quantification was measured by mean fluorescence intensity. Data represented for all confocal microscopy studies (phagocytosis, LC3B-BCG colocalization and p62-BCG colocalization) as mean values ± S.E.M. (n= 3 independent biological replicate experiments). All statistical analyses done using two-tailed Student’st-test (*P< 0.05, **P< 0.01, ***P< 0.001, ****P< 0.0001). Data shown are for BCG-Tice; similar findings were observed for BCG-Pasteur as shown in Figs.S2andS7. Tumor weight measurement, macrophage, and lymphocyte quantification done using two-tailed Student’s t -test (* P < 0.05, ** P < 0.01, *** P < 0.001, **** P < 0.0001). Full size image To confirm the STING pathway dependence of these antitumor and cellular immunologic changes elicited by BCG- disA -OE, we repeated the above MB49 tumor experiments in STING −/− mice as outlined in Fig. S15a . Mean tumor weights in MB49-inoculated STING −/− mice were 0.7 g at following BCG- disA -OE treatment (not significantly different from untreated WT or untreated STING −/− mice) whereas it was 0.2 g in treated WT mice (P = 0.02) (Fig. S15b ) and this was associated with an overall reduction of immune (CD45 + ) cells infiltrating tumors in STING −/− mice as compared with WT mice (Fig. S15c ). Among tumor-infiltrating lymphocytes, there were large reductions in total lymphocytes and activated CD8 + T cells (IFN-γ + CD8 cells, CD25 + CD69 + CD8 cells, and CD69 + CD38 + CD8 cells) in tumors from treated STING −/− mice compared with WT mice, changes that were less pronounced in untreated or BCG-WT treated STING −/− and WT mice (Fig. S15d–g ). Likewise, activated tumor-infiltrating macrophages (TNF-α + F4/80 + CD11b + cells and TNF-α + CD206 + CD124 + ) were notably reduced in BCG- disA -OE-treated STING −/− mice compared with WT mice (Fig. S15h, i ). These findings confirm that the antitumor effects of BCG- disA -OE are largely STING-dependent. Safety: BCG- disA -OE is less pathogenic than BCG-WT in two mouse models To address concerns that the enhanced pro-inflammatory immune responses elicited by BCG- disA -OE might lead to adverse effects, we evaluated safety in two separate mouse models. We used an immunocompetent BALB/c mouse model of aerosol exposure and measured the lung bacillary burden after 4 weeks when adaptive immune responses are maximal (Fig. 7a ). While the day 1 implantation of the two BCG strains was equivalent, we observed that BCG- disA -OE proliferated in murine lungs to a significantly lower degree than BCG-WT by a margin of 0.43 log 10 colony forming units (Fig. 7b and Fig. S16a ). As we observed in earlier in cell-based models, pro-inflammatory cytokine levels in both lungs and spleens were significantly higher in BCG- disA -OE-exposed mice than those receiving BCG-WT (Fig. 7c, d and Fig. S16b ). We also tested the two strains in immunocompromised SCID mice, which do not survive infection with BCG. Again, using a low-dose aerosol exposure model (Fig. 7e ), we observed a statistically significant survival prolongation with BCG- disA -OE compared to BCG-WT (Fig. 7f and Fig. S16c ). Thus, despite eliciting more profound inflammatory signatures in numerous model systems, BCG- disA -OE is less pathogenic than BCG-WT in these two murine model systems. Fig. 7: BCG- disA -OE is less pathogenic than BCG-WT in two mouse models and elicits a greater pro-inflammatory cytokine levels in vivo. a Schematic diagram of the immunocompetent BALB/c mouse challenge model. b Lung colony forming unit (CFU) counts at day 1 ( n = 3 animals/group) and day 28 ( n = 5 animals/group). Data are represented as mean values ± S.E.M. c Levels of the pro-inflammatory cytokines IFN-β, TNF-α, IL-6, and IFN-γ in mouse lungs and d spleens determined by ELISA at day 28 ( n = 4 animals/group). Data are mean values ± S.E.M. e Schematic diagram of the immunocompromised SCID mouse challenge model. f Percent survival of SCID mice following low-dose challenge ( n = 10 animals/group). The day 1 lung CFU counts are shown at right ( n = 2 animals/group). All statistical analyses done using two-tailed Student’s t -test (* P < 0.05, ** P < 0.01, *** P < 0.001, **** P < 0.0001). Full size image Numerous recombinant BCG strains have been generated and tested over the years. These studies were generally conducted with the goal of improving either TB protective efficacy or bladder cancer immunotherapy, but in certain cases the goal has been prevention of other infectious diseases [45] , [46] . A common strategy has been to overexpress an antigen to elicit disease-specific immunity or a cytokine gene to boost local host responses [47] , [48] . While many modified BCGs have shown efficacy in pre-clinical models, few have progressed to human clinical trials. To date only BCGΔ ureC :: hly (VPM1002), a BCG designed to enhance phagosome permeability and exposure of BCG antigens to cytosolic MHC class I antigen processing [49] , has advanced to late stage clinical trials for tuberculosis [50] . The innovative aspect of our study is to specifically re-engineer BCG with the goal of improving trained immunity by overexpressing the PAMP molecular cyclic-di-AMP, thereby amplifying STING pathway engagement. The primary goal of this study was to determine whether heterologous immune responses-or so-called trained immunity-elicited by BCG can be modulated. As BCG is currently a candidate vaccine for COVID-19 [3] , [4] and is being considered for other uses such as protection against infections in the elderly [2] and improved glycemic control in diabetes [51] , addressing this question is clinically relevant. As it has been postulated that combinations of vaccines may be necessary to protect a sufficient fraction of the population against COVID-19 [52] , knowledge of whether vaccine candidates such as BCG may be potentiated is important. As trained immunity results from engagement of PRRs by pathogen-generated PAMPS, we generated a recombinant BCG that overexpresses cyclic-di-AMP, a PAMP expressed in low levels by a number of pathogens. 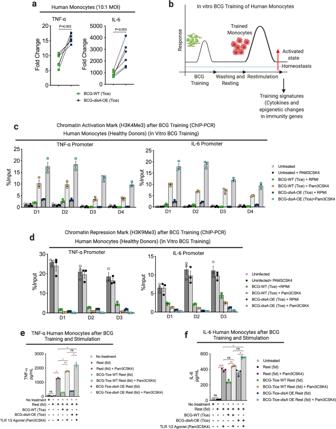Fig. 3: Compared with BCG-WT, BCG-disA-OE is a more potent inducer of epigenetic changes characteristic of trained immunity in primary human monocytes. amRNA levels of TNF-α and IL-6 in primary human monocytes (n= 6 healthy donors) relative to RNU6A after 24 h exposures at a MOI of 10:1. Statistical analysis done using multiple unpaired t-test with Bonferroni-Dunn method.bSchematic diagram of in vitro monocyte training.cRelative levels of the H3K4me3 chromatin activation mark (n= 4 healthy donors; D1–D4) ordthe H3K9me3 chromatin repression mark retrieved from TNF-α and IL-6 promoter regions of primary human monocytes from 3 (n= 3) health donors (D1–D3) determined by ChIP-PCR assay on day 6.e,fSecreted cytokines (TNF-α and IL-6) following BCG training and re-stimulation. Monocytes were initially challenged on day 0 with a 24 h exposure to the BCG strains at a MOI of 10:1 followed by washing. After 5 days of rest, they were treated for 24 h with either a sham stimulus (RPMI) or the TLR1/2 agonist Pam3CSK4 (n= 3 healthy donors). Data are presented as mean values ± S.E.M. Statistical analyses done using two-tailed Student’st-test (*P< 0.05, **P< 0.01, ***P< 0.001, ****P< 0.0001). Cyclic-di-AMP is recognized by the host PRR, STING, and via the TBK1/IRF3 pathway leads to increased expression of Type 1 interferons and subsequent recruitment of activated T cells [23] . Because of its role in elevating Type 1 interferon levels, STING pathway activation has been proposed as a non-specific antiviral strategy and is being tested against COVID-19 in pre-clinical models [53] . To determine if trained immunity parameters may be increased, we tested BCG- disA -OE versus BCG-WT in a battery of in vitro assays. We evaluated cytokine release profiles, macrophage polarization, autophagy, phagocytosis, epigenetic modifications, and metabolic remodeling in human and murine primary cells. In each assay system, BCG- disA -OE was a more potent potentiator of pro-inflammatory responses than BCG-WT. We further tested the cyclic-di-AMP expressing BCG in a functional in vivo assay of trained immunity, namely bladder cancer immunotherapy. In two separate models of urothelial cancer, BCG- disA -OE has greater immunotherapeutic efficacy than did BCG-WT indicating that our in vitro results were predictive of functional efficacy in a relevant animal model. Interestingly, despite eliciting a significantly more potent pro-inflammatory responses in our in vitro assay systems, BCG- disA -OE did not produce excess pathogenicity in two animal models of BCG infection or BCGosis [54] . We also observed that BCG-WT did not uniformly elicit pro-inflammatory responses. For example, we observed that treatment of murine macrophages with BCG-WT in fact induced a higher percentage of M-MDSCs (anti-inflammatory) compared with untreated controls (Fig. 2a ), and similarly BCG-WT led to elevated levels of the anti-inflammatory metabolite kynurenine (Fig. 4a ). These findings of certain anti-inflammatory consequences of BCG-WT may correlate with the observation that in countries that routinely use BCG for TB prevention, vaccinees display reduced levels of asthma and atopic dermatitis [55] , [56] . In contrast, this expansion of M-MDSCs in macrophages by BCG-WT was reversed by cyclic-di-AMP overexpression, which is in keeping with a recent study showing that STING pathway activation reduces the induction of MDSCs in certain cancers [57] . Trained immunity changes elicited by BCG may underlie the immunotherapeutic effects of BCG in cancer prevention [40] . Therefore, another goal of this study was to evaluate whether the salutary effects of BCG- disA -OE as a NMIBC immunotherapy is mediated through engagement of STING pathway and modulates BCG-mediated trained immunity. In a rat model of NMIBC, we found that whereas invasive tumors developed in untreated tumor-bearing rats (highest tumor grade of T2) as well as BCG-WT-treated animals (highest tumor grade of T1), invasive bladder cancer was completely absent in rats treated with BCG- disA -OE. Similarly, in the MB49 mouse model of bladder cancer, BCG- disA -OE was superior to BCG-WT in reducing tumor growth with associated increase in tumor necrosis, and these effects were accompanied by significantly higher recruitment of activated, inflammatory macrophages, IFN-γ-producing CD4 T cells, and reduced accumulation of Treg cells in the tumors. In STING −/− mice these antitumor effects and immunologic changes were absent indicating that the activity of BGC- disA -OE is STING-dependent. We observed elevated levels of pro-inflammatory cytokines and chemokines in bladders from tumor-bearing animals treated with BCG- disA -OE compared to BCG-WT. Since non-immune cells have also been shown to possess immunological memory [58] , we considered the possibility that this cytokine response may have originated from myeloid cells in the TME and/or the tumor cells themselves. Indeed, we found that compared with BCG-WT, BCG- disA -OE elicited more potent cytokine responses in both primary macrophages and human urothelial cancer cells representing various tumor stages, though it remains formally possible that the other cells such as bone-marrow progenitors may contribute to BCG-mediated immune responses as has been reported [9] , [59] . These heightened cytokine and cellular immune responses observed with BCG- disA -OE appear to be a downstream consequence of STING activation since we found dramatically reduced cytokine expression in BMDMs from STING −/− mice and in activated CD8 T cells and macrophages infiltrating MB49 tumors in treated STING −/− mice. In addition, we found robust induction of several chemokines in rat bladders treated with BCG- disA -OE as has been observed in other studies with stimulation using exogenous STING agonists [19] , [60] . Our results support the conclusion that BCG-mediated trained immunity can be increased by elevated production of a relevant PAMP and STING pathway engagement. This suggests that efforts to utilize BCG clinically for COVID-19 vaccination, infection reduction the elderly, NMIBC, and tuberculosis should consider the strategy of PAMP overexpression and utilize trained immunity markers as a pre-clinical development milestone. Ethics All protocols involving animals strictly adhered to US NIH guidelines and were approved by the Johns Hopkins Medical Institutions Animal Care and Use Committee under the protocols: MO18M58, MO20M20, and RA17M332. Bacterial strains and culture conditions In this study we used Mycobacterium bovis ( M. bovis ) Bacillus Calmette- Guérin (BCG) Pasteur (BCG-WT Pasteur) (a generous gift from Dr. Frank Collins [FDA] and identical to BCG-Pasteur provided by the Pasteur Institute to the Trudeau Institute in 1967 as TMC No. 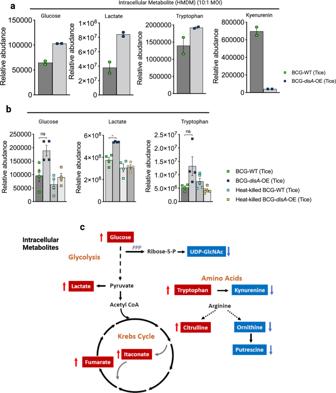Fig. 4: Compared with BCG-WT, BCG-disA-OE is a more potent inducer of metabolomic changes characteristic of trained immunity in primary human monocytes. a,bMetabolite levels determined by LC-MS in human (n= 2 independent biological replicate), or murine MDM (n= 4 independent biological replicate experiments) determined 24 h after exposure to BCG strains or heat-killed controls. The data are presented as mean values ± S.E.M. Cartoon diagramcshowing key metabolites significantly upregulated (red arrow upward) or downregulated (blue arrow downward) in BCG-disA-OE infected macrophages relative to BCG-WT infected macrophages. Statistical analyses done using two-tailed Student’st-test (*P< 0.05). 1011) and commercially available BCG-Tice (Onco-Tice © , Merck) for for generation of c-di-AMP overexpressing recombinant BCG strains. Briefly, genomic DNA from Mycobacterium tuberculosis ( M. tb ) strain CDC1551 was used for PCR amplification of disA (MT3692/Rv3586). Single isolated bacterial colonies growing on 7H11 plates supplemented with oleic-albumin-dextrose-catalase (OADC) (Cat. B11886, Fisher Scientific) were picked and propagated in 7H9 Middlebrook liquid medium (Cat. B271310, Fisher Scientific) supplemented with (OADC) (Cat. B11886, Fisher Scientific), 0.5% glycerol (Cat. G55116, Sigma) and 0.05% Tween-80 (Cat. BP338, Fisher Scientific). Cloning experiments were performed using E. coli strain DH5-α (Cat. 18258012, Fisher Scientific) and was routinely maintained in LB broth. For generation of disA overexpressing BCG, an E. coli -mycobacterial shuttle vector (pSD5.hsp60) was used to clone M.tb gene MT3692 or Rv3586 under the strong mycobacterial promoter hsp60 . Clones were confirmed by gene sequencing and were used for bacterial transformation by electroporation method. Recombinant strains were confirmed using colony PCR against kanamycin cassette, subjected to whole genome sequencing and qPCR analyses. Details of all bacterial strains, plasmids and constructs are listed in Supplementary Table S1 . Mammalian cell culture Cell lines For cell-based in vitro infection assays J774.1 (American Type Culture Collection-ATCC® TIB67™, Manassas, VA, USA) murine macrophage cell lines were cultivated in RPMI-Glutamax (Cat. 61870-036, Fischer Scientific), supplemented with 10% heat inactivated fetal bovine serum (FBS) (Cat. 10082147, Fischer Scientific) with 1% streptomycin/penicillin at 37 °C with 5% CO 2 . Urothelial carcinoma cell lines 5637 (ATCC® HTB-9™), a human high-grade urothelial cancer; RT4 (ATCC ® HTB-2™), a human transitional cell low-grade urothelial cancer; J82 (ATCC® HTB-1™), a human high-grade urothelial cancer; and NBT II (ATCC® CRL-1655™), N-butyl-N-(4-hydroxybutyl) nitrosamine induced tumor cell line in Rattus norvegicus Nara Bladder Tumor No. 2, UPPL1595 (luminal cell line established from a spontaneous primary bladder tumor in an Uroplakin-Cre driven PTEN/P53 knockout genetically engineered mouse model and were generously provided by Dr. William Kim (UNC Chapel Hill)., BBN975 (basal- cell line established from, 0.05% N-Butyl-N-(4-hydroxybutyl) nitrosamine (BBN) induced murine urothelial cancer model and was generously provided by Dr. William Kim (UNC Chapel Hill), and MB49 (murine urothelial carcinoma cells, 7,12-dimethylbenz[a]anthracene (DMBA, EMD Millipore, Cat. SSC148) were maintained as monolayer in RPMI1640 medium supplemented with 10% heat inactivated fetal bovine serum (FBS) with 1% streptomycin/penicillin at 37 °C with 5% CO 2 . Mouse fibroblast cell line NCTC clone 929 [L cell, L-929, derivative of Strain L] (ATCC® CCL-1™) were routinely maintained as monolayer in DMEM media supplemented with 10% heat inactivated fetal bovine serum (FBS) with 1% streptomycin/penicillin at 37 °C with 5% CO 2 . All cell lines were not maintained more than 10 passage cycle and Mycoplasma testing was performed periodically while cells were in culture. Reporter mouse cell line, RAW-Lucia ISG (InvivoGen, CA, USA) was cultivated in custom prepared media as per manufacturer’s instructions. Primary cells (macrophages and dendritic cells) For generation of murine bone-marrow-derived macrophages (BMDMs) and dendritic cells (BMDCs), bone-marrow (BM) cells were isolated from 4-week-old female wild-type (WT) C57BL/6J (Charles River laboratories, North Wilmington, Mass) and STING-KO mice (C57BL/6J-Tmem173gt/J, Jackson laboratories). The seed stock containing multiple vials of bone-marrow cells were preserved in cryopreservation media containing 10% DMSO (Cat. D2650; Sigma) and 90% heat inactivated FBS (Cat. 10082147, Fischer Scientific) in liquid nitrogen. For differentiation of BM cells into macrophages or DCs, random cryopreserved vials were chosen and differentiated for 6 days in BMDM-differentiation media made from DMEM containing 10% FBS, 1% MEM amino acids (Cat. 11130051, Thermo Fisher Scientific), 1% MEM non-essential amino acids (Cat. 11140050, Thermo Fisher Scientific), 1% sodium pyruvate (Cat. 11360070, Thermo Fisher Scientific), 1% MEM vitamin (Cat. 11120052, Thermo Fisher Scientific) and antibiotics (Penicillin-Streptomycin solution) supplemented with 30% sterile mouse fibroblast L929 (ATCC® CCL-1™) conditioned media. Differentiation of BM cells into DCs was carried out in low attachment 10 mm cell culture dish in presence of bone-marrow-differentiation media in presence of recombinant murine Granulocyte-Macrophage Colony-Stimulating Factor (GM-CSF) (Cat. 315-03, Peprotech) for 48 h. Non-adherent cells were washed and loosely attached cells were allowed to differentiate into BMDCs for next 6 days. Cells were characterized for macrophage and DC markers using cell-surface staining and flow-cytometry analyses. Human primary monocytes and human monocyte-derived macrophages (HMDMs) were used for cell-based in viro infection assays. Peripheral blood-derived mononuclear cells (PBMCs) isolated from healthy male donors (leukopacks) aged between 18-30 were used for isolation of human monocytes (HM) or human monocyte-derived macrophages (HMDM). Briefly, to separate blood constituents and isolation of buffy coat density gradient centrifugation (400 × g at 18 °C for 30 min) of RPMI-1640 diluted blood over a Ficoll-Paque™ Plus reagent (Cat. 17-1440-02, GE Healthcare, Piscataway, NJ) was performed. Cells were washed several times using 1x phosphate-buffered saline (PBS) and were counted using hemocytometer. Once counted CD14 + human monocytes were isolated from PBMCs using magnetic labeling (Monocyte Isolation Kit II, Cat. 130-091-153, Miltenyi Biotec, San Diego, CA) and magnetic columns as per manufacturer’s instructions. The purity of isolated CD14 + cells was confirmed using a fraction of cells stained with a fluorochrome-conjugated antibody against a monocyte marker as recommended by manufacturer and cells were analyzed using BD-LSR2 flow cytometer. Human monocytes were seeded (2.0–3.0  × 10 5 cells/ml in RPMI 1640 medium supplemented with 10% FBS and 1% streptomycin/penicillin at 37 °C with 5% CO 2. Monolayers of CD14 + monocytes were differentiated into M1 [GM-CSF (20 ng/ml, PeproTech, Rocky Hill, NJ) and IFN-γ (20 ng/ml, PeproTech, Rocky Hill, NJ PeproTech)] or M2 [M-CSF (20 ng/ml, PeproTech, Rocky Hill, NJ) and IL-4 (20 ng/ml, PeproTech, Rocky Hill, NJ PeproTech)] for next 7 days. Animals Experimental procedures involving live animals were carried out in agreement with the protocols approved by the Institutional Animal Care and Use Committee (IACUC) at The Johns Hopkins University School of Medicine. For animal infection protocols, pathogen-free age 4–6 weeks female C57BL/6J (Charles River Laboratories, North Wilmington, Mass. ), C57BL/6J-Sting1<gt>/J (STING −/− Golden ticket mouse) (The Jackson Laboratory, ME, US), Fox Chase SCID mice (Charles River Laboratories North Wilmington, Mass.) and BALB/c mice (Charles River Laboratories, North Wilmington, Mass.) were purchased and housed under pathogen-free conditions at an Animal Biosafety Level-3 (ABSL3) or Biosafety Level-2 (ABSL2) animal facility without cross-ventilation. Fischer 344 female rats age 8 weeks (Harlan, avg. weight 160 g) were housed at an BSL2 animal facility. Animals were housed under standard housing conditions (68–76 °F, 30–70% relative humidity, 12–12 light-dark cycle) with free access to water and standard chow and were monitored daily for general behavior and appearance by veterinary specialists. In vitro infection assays For in vitro infection assays, cell lines or primary cells were seeded at required cell density in 6-well tissue culture plates or 10 mm petri dishes. For infection, log-phase wild-type and BCG- disA -OE strains were harvested by centrifugation and washed twice using DPBS to remove residual detergent and BSA then suspended in antibiotic-free RPMI 1640 media supplemented with 10% FBS. For infection assays, the bacteria were deposited at pre-calibrated multiplicity of infection (MOI). Infection was allowed for next 4 h, followed by repeated washing of infected cells using warm DPBS to remove non-internalized bacteria. Infected cells were incubated until endpoints in presence of RPMI-1640 medium supplemented with 10% FBS and antibiotics. Toxicity assays Human urothelial cancer cell lines, RT4, 5637, and J82, were cultured at 37 °C under 5% CO 2 in RPMI 1640 containing 10% FBS without antibiotics. For cell toxicity assay, 3000 cells for RT4 and 1500 cells for 5637 and J82 were seeded in a 96-well tissue-treated plate in triplicate, respectively. Twenty-four hours after seeding, cells were treated with the indicated ratio of BCG to cells for 72 h. To measure cell viability, CellTiter-Glo Luminescent Cell Viability Assay (Promega, Madison, WI, USA) and FLUOstar OPTIMA (BMG Labtech, Ortenberg, Germany) were used according to manufacturer’s protocols. Relative cell viability was calculated by dividing the viability of the indicated ratio by that of a control. For Annexin-PI staining, 0.5 million J774.1 cell and BMDMs were plated per well in 6-well plates for physical attachment. Cells were exposed at 1:10 MOIs for 24 h using wild-type and BCG- disA -OE strains of Tice and Pasteur to determine the BCG cytotoxicity following exposure. At the endpoint of infection or treatment cells were non-enzymatically removed using 0.02% EDTA-PBS solution. Cells were washed twice with ice-cold PBS and FITC-annexin-PI was done as per manufacturer’s instruction using FITC-Annexin V Apoptosis Detection Kit I (Cat. 556547, BD Biosciences). Flow-cytometry was performed using a BD LSRII flow cytometer of the Flow Cytometry Core Facility at The Bloomberg School of Public Health, Johns Hopkins University). Data was processed using FACSDiva (v 9.0) and FlowJo (Tree Star v10) softwares. Quantitative real-time qPCR Gene expression profiling was carried out using total RNA isolated from cell lines or primary cells. For RNA isolation from rat bladders, pieces of whole bladder samples were excised, snap-frozen in liquid nitrogen immediately after harvesting and stored in RNAlater (Cat. AM7021, Ambion) at –80 °C. Total RNA isolation was carried out using RNeasy system (Cat. 74106, Qiagen). Real-time qPCR was performed using the StepOnePlus system (Applied Biosystems). For gene expression analyses in cell lines and primary cells, SYBR Fast green double stranded DNA binding dye (Cat. 4085612, Applied Biosystems) was used. Gene expression analyses in rat bladder tissues were performed using TaqMan gene expression assays. Gene-specific qPCR primers were purchased from Integrated DNA Technologies and all TaqMan gene expression assays were purchased from Thermo Fischer Scientific. Amplification of RNU6a, β-actin, GAPDH were used as endogenous control for RNA samples derived from human, mouse and rat cells/tissues respectively. All experiments were performed at least in triplicate and data analyses was done using 2 −∆∆CT method. Details of NCBI gene identifiers and primer sequences are given in the supplementary table S2 . Enzyme-linked immunosorbent assay (ELISA) Sandwiched ELISA was performed for cytokine (IFN-β, TNF-α, IL-6, IFN-γ, IL-1β and MCP-1/CCL2) measurement in culture supernatants and animal tissues from lung, spleen or urinary bladder. Briefly, tissues and culture supernatants were flash frozen in liquid nitrogen immediately after harvest and stored at –80 °C. Animal tissues were homogenized using micro tissue homogenizers (Cat. 1215D61, Kimble) and filter sterilized for measurement of various cytokine protein expression levels using sandwiched ELISA as per manufacturer’s recommendations. Details of all ELISA kits and accessory reagents are given in Supplementary Table S2 . Multicolor confocal microscopy Multicolor laser confocal microscopy experiments were performed to determine phagocytosis, autophagy, and colocalization studies in urothelial cancer cells and primary macrophages. Briefly, cells were allowed to adhere on sterile glass cover slips placed in 6-well tissue culture plates and infections were carried at pre-calibrated MOI. Log-phase bacterial cultures were labeled using FITC (Cat. F7250, Sigma). Following infection and treatment conditions, cells were fixed, permeabilized and blocked followed by overnight incubation with a primary antibody for LC3B (Cat. NB100-2220, Novus) or p62/SQSTM1 (Cat. P0067, Sigma-Aldrich) at recommended dilutions at 4 °C. Cells were washed and incubated in the dark with Alexa Flour 647 conjugated secondary antibody (Cat. A32733, Thermo Fisher Scientific) at 4 °C for 1 h. DNA staining was carried out using Hoechst 33342 (Cat. 62249, Thermo Fisher Scientific) for 5 min. Images were acquired using Zeiss LSM700 single-point, laser scanning confocal microscope at x63 magnification at the Microscope Facility, Johns Hopkins School of Medicine. Image processing and analyses was carried out using open-source Fiji software ( https://imagej.net/software/fiji/ ). For LC3B or p62 quantification, perinuclear LC3B puncta (spot) was counted in a minimum 100 cells across different fields using and Imaris 9.5.0. Quantification carried out using GraphPad Prism (Prism 9.0) software. Phagocytosis assay IgG-FITC conjugated latex bead phagocytosis assay kit (Item No. 500290, Cayman Chemicals, USA) was used for phagocytosis studies. Briefly, HMDMs were placed on sterile glass cover slip for attachment. Infection was carried out at 5:1 (HMDM versus BCG) ratio for 3 h followed by addition of IgG-FITC beads in warm RPMI 1640 media at 1: 400 dilutions for 3 h. Nuclear staining was carried out using Hoechst 33342 (Cat. 62249, Thermo Scientific) and cells were visualized for bead phagocytosis using Zeiss LSM700 single-point, laser scanning confocal microscope. Quantification of beads was measured by mean fluorescence intensity (M.F.I.) calculations using open-source Fiji Software ( https://imagej.net/software/fiji/ ). Multicolor flow cytometry The cell surface and intracellular staining was carried out on J774.1, murine BMDMs, human HMDMs and single cells derived from murine MB49 tumors and spleens. Flow-cytometry panel were designed and if needed modified form murine myeloid and lymphoid cells and human myeloid cells. Details of all antibodies and the dilutions used are given in the Supplementary Table S2 . For in vitro infection assays, protein transport inhibitor cocktail (Cat. 00-4980-03, eBioscience) at recommended dilution, 12 h before harvesting monolayer of cells. At the endpoint cells were harvested using a cell-detachment buffer (ice-cold PBS-10 mM EDTA solution). Single-cell isolation was performed using animal tissues by harvesting tumors and spleens following necropsy. Briefly, tissues were manually disrupted before incubating in collagenase type I (Gibco) and DNase (Roche) in RMPI for 30 min at 37 °C. Tumor and spleen cells were dissociated through a 70-μm filter and washed with PBS. RBC lysis was performed for 5 min using ACK lysis buffer (Cat. A1049201, Thermo Fisher Scientific) at room temperature. Cells were washed twice using ice-cold PBS and stained using Zombie Aqua™ Fixable Viability Kit (Cat. 423101, Biolegend). Cells were washed and resuspended in FACS buffer (1% BSA, 2 mM EDTA in PBS), Fc blocked (TruStain FcX™, Cat. 101320, and True-Stain Monocyte Blocker™ Cat. 426102 Biolegend) and stained with conjugated primary antibodies as per manufacturer’s protocol and pre-titrated antibody dilutions (Supplementary Table S1 ). Intracellular staining was performed following fixation and permeabilization (Fixation and Permeabilization Buffer Set, eBioscience). Cells were washed and resuspended in flow buffer and acquired using BD LSRII with FACSDiva Software (v 9.0). analyses were performed using FlowJo (v10) (TreeStar). The following antibodies were used to stain myeloid and lymphoid cells: Mouse BMDMs: Anti-CD45 (clone 30-F11), anti-CD124 (clone I015F8), anti-I-A/I-E (clone 107630), anti-Ly6C (clone HK1.4), anti-CD11b (clone M1/70), anti-F4/80 (clone BM8), anti-Ly6G (clone 1A8), anti-CD206 (clone C068C2), anti-TNF (clone MP6-XT22) all Biolegend), anti- IL-10 (clone JES5-16E3 eBiosciences), and anti-Glut1 (clone EPR3915, Abcam). Human HMDMs: anti CD16 (clone 3G8), anti-CD14 (clone 63D3), anti-HLA-DR (clone L243), anti-CD11b (clone ICRF44), anti-CD206 (clone 15-2), anti-CD163 (clone GHI/61), anti-TNF (clone MAb11), and anti-TNF (clone MAb11) all Biolegend. Mouse macrophages (syngeneic MB49 model of urothelial carcinoma): CD45 (clone 30-F11, Biolegend), CD124 (IL-4Ra) (clone I015F8, Biolegend), I-a/I-e (clone M5/114.15.2, Biolegend), F4/80 (clone BM8, Biolegend), CD206 (clone C068C2, Biolegend), TNF (clone MP6-XT22, Thermo Fisher), IL-10 (clone JES5-16E3, Thermo Fisher). Mouse T cells (syngeneic MB49 model of urothelial carcinoma): CD45 (clone PerCP, Biolegend), CD25 (clone PC61, Biolegend), CD3 (clone 17A2, Biolegend), CD4 (clone GK1.5, Biolegend), CD8a (clone 53-6.7, Biolegend), FOXP3 (clone MF-14, Biolegend), Mouse IFN-γ (clone XMG1.2, Biolegend) and FOXP3 (clone MF-14 Biolegend), CD69 (cloneH1.2F3, Biolgened), CD38 (clone IM7, Biolegend). In vitro monocyte trained immunity experiment In vitro training of primary human monocytes was performed according to the well-established model [33] . Briefly, PBMCs were isolated from healthy donors (leukopaks). Following magnetic separation, CD14 + monocytes were seeded in 10 mm tissue culture dishes for 3 h in warm RPMI 1640 media supplemented with 10% FBS at 37 °C with 5% CO 2 . Non-adherent cells were removed by washing cells using warm PBS. Monolayer culture of human monocytes was infected with BCG-WT and BCG- disA -OE strains at 5:1 (monocyte versus BCG) MOIs for 4 h in the presence of RPMI 1640 supplemented with 10% FBS. Non-internalized bacilli were washed out using warm PBS and subsequently incubated for 24 h. Cells were again washed using warm PBS and fresh warm RPMI 1640 media was added. For the following 5 days, cells were allowed to rest with a PBS wash and addition of fresh media every second day. Cells were re-stimulated on day 6 with RPMI 1640 supplemented with 10% FBS (negative control, without training) or TLR1/2 agonist, Pam3Cys (Cat. tlrl-pms, InvivoGen). Following stimulation, for 24 h, culture supernatants were collected, filter sterilized and quickly snap-frozen (–80 °C) for cytokine measurement. Cells were harvested for chromatin immunoprecipitation (ChIP) experiments to measure epigenetic changes on gene promoters. Chromatin immunoprecipitation (ChIP) Human monocytes were fixed with a final concentration of 1% formaldehyde for 10 min at room temperature. Cell fixation was stopped using 125 mM glycine (Cat no. 50046, Sigma-Aldrich, USA), followed by sonication to fragment cellular DNA to an average size between 300 to 600 bp using Qsonica Sonicator Q125 (Cat. 15338283, Thermo Fisher Scientific). Sonicated cell lysates were subjected to immunoprecipitation (IP) by overnight incubation with recommended concentration of primary antibodies [(Histone H3K9me3 (H3K9 Trimethyl) Polyclonal Antibody cat. A-4036-100, epigentek); Anti-Histone H3 (trimethyl K4) antibody-ChIP Grade (ab8580), abcam)] in presence of magnetic Dynabeads (Cat no. 10004D, Thermo Fisher Scientific, USA) at 4 °C. Non-bound material was removed by sequentially washing the Dynabeads with lysis buffer, chromatin IP (ChIP) wash buffer and Tris-EDTA (TE buffer). DNA elution was done using ChIP elution buffer. Amplification of different segments of the regulatory regions of immunity genes was carried out using qPCR using specific primers. Reactions were normalized with input DNA while beads served as negative control. Details of all primary antibodies and sequence of primers have been given in Supplementary Table. S2 . Targeted metabolite analysis with LC-MS/MS Targeted metabolite analysis was performed with liquid-chromatography tandem mass spectrometry (LC-MS/MS). Metabolites from cells were extracted with 80% (v/v) methanol solution equilibrated at –80 °C, and the metabolite-containing supernatants were dried under nitrogen gas. Dried samples were resuspended in 50% (v/v) acetonitrile solution and 4 ml of each sample were injected and analyzed on a 5500 QTRAP triple quadrupole mass spectrometer (AB Sciex) coupled to a Prominence ultra-fast liquid-chromatography (UFLC) system (Shimadzu). The instrument was operated in selected reaction monitoring (SRM) with positive and negative ion-switching mode as described. This targeted metabolomics method allows for analysis of over two hundred of metabolites from a single 25-min LC-MS acquisition with a 3-ms dwell time and these analyzed metabolites cover all major metabolic pathways. The optimized MS parameters were: ESI voltage was +5000 V in positive ion mode and –4500 V in negative ion mode; dwell time was 3 ms per SRM transition and the total cycle time was 1.57 s. Hydrophilic interaction chromatography (HILIC) separations were performed on a Shimadzu UFLC system using an amide column (Waters XBridge BEH Amide, 2.1 × 150 mm, 2.5 μm). The LC parameters were as follows: column temperature, 40 °C; flow rate, 0.30 ml/min. Solvent A, Water with 0.1% formic acid; Solvent B, Acetonitrile with 0.1% formic acid; A non-linear gradient from 99% B to 45% B in 25 min with 5 min of post-run time. Peak integration for each targeted metabolite in SRM transition was processed with MultiQuant software (v2.1, AB Sciex). The preprocessed data with integrated peak areas were exported from MultiQuant and re-imported into Metaboanalyst software (MetaboAnalyst (V5.0) ( https://www.metaboanalyst.ca ) for further data analysis including statistical and principal component analyses. Glucose uptake assay Glucose uptake measurement was performed on bone-marrow-derived macrophages (BMDMs) isolated from C57BL/6 females in an in vitro BCG infection assay. Briefly, macrophages were infected at a ratio of 1:20 (macrophage vs. BCG-WT or BCG- disA -OE) in presence of DMEM medium devoid of glucose for 4 h. Exogenous addition of 2-NBDG was carried out and cells were stained for cell surface markers (Glut1 and CD45) after 2 h of incubation. Expression of Glut1 expression and 2-NBDG positivity was determined using flow-cytometry analyses using FACSDiva (v 9.0) and FlowJo (v10) (TreeStar). Histologic analyses and immunohistochemistry (IHC) For histologic analyses, a portion of bladder was formalin fixed and paraffin embedded. Sections of 5 μ in thickness on glass slides were stained with hematoxylin-eosin for classification according to the World Health Organization/International Society of Urological Pathological consensus. Tumor staging was performed by two board-certified genitourinary pathologists (A.S.B., A.M.) blinded to treatment groups. Specimens were classified based on the percentage of involvement of abnormal tissue (1 = 10% involvement, 2 = 20% involvement, and so forth). For IHC staining, high-temperature antigen retrieval (18–23 psi/126 °C) was performed by immersing the slides in Trilogy (Cell Marque). Endogenous peroxidase activity was blocked for 5 min in using Dual Endogenous Enzyme Block (Cat. S2003, Dako). Primary Antibodies used included Ki67 (1:50, Cat. ab16667; Abcam), CD68 (1:250, Cat. MCA341R; Serotec), CD86 (1:100, Cat. bs-1035R; Bioss) and CD206 (1:10 K, Cat. ab64693; Abcam). For Ki67, slides were stained with ImmPACT DAB (Vector Labs) for 3 min and counterstained with haematoxylin (Richard-Allen). Dual staining for CD68/CD206 and CD68/CD86 was achieved by first staining for CD68 with Impact DAB (Vector Labs) followed by secondary antigen retrieval and incubation as above with either CD86 or CD206 and visualized with ImmPACT AEC (Vector Labs). For each section, Ki67 expression was scored as a percentage of positive cells in the urothelium. Dual stains for CD68/CD86 and CD68/CD206 were scored based on positive clusters of cells for each marker (0 = no staining, 1 = rare isolated cells positive, 2 = clusters of up to 10 positive cells, 3 = clusters of >10 positive cells). In vivo experiments Intravesical BCG treatment in carcinogen-induced NMIBC rat model The induction of urothelial cancer in rats and subsequent treatment of intravesical BCG were carried out using our published protocol. Briefly, N-methyl-N-nitrosourea (MNU) instillations were given every other week for a total of four instillations. Fischer 344 female rats age 7 weeks (Harlan, avg. weight 160 g) were anesthetized with 3% isoflurane. 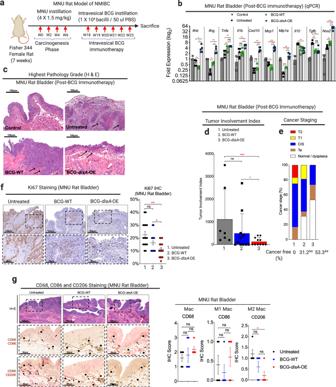Fig. 5: BCG-disA-OE elicits improved antitumor efficacy over BCG-WT in the orthotopic carcinogen-induced rat model of urothelial cancer. aSchematic diagram of the MNU rat model of NMIBC.bmRNA levels for pro-inflammatory cytokines (Ifnb,Ifng,Tnfa, andIl1b), regulatory chemokines (Cxcl10,Mcp1, andMip1a), immunosuppressive M2-like macrophage cytokines (Il10andTgfb) and M1-like tumoricidal effectors (Nos2) in whole bladders at necropsy (wk 23) measured by qRT-PCR relative to GAPDH (n= 5 animals/group).cRepresentative H&E staining showing highest pathology grade for each group [control, untreated MNU bladder, BCG-WT (Past and Tice), and BCG-disA-OE (Past and Tice) (n= 12–16 animals/group)].dTumor involvement values at necropsy (7–11 animals/group).eHighest tumor stage at necropsy.fRepresentative immunohistochemistry and bar graph of rat bladder tissue at necropsy stained for Ki67 (n= 17–22 animals).gRepresentative immunohistochemical co-staining and line graph for CD68 (brown), CD86 (M1-like macrophages; red) and CD206 (M2-like macrophages; red) in rat bladder tissues at necropsy (n= 5 animals per group). Data are presented as mean values ± S.E.M. (qRT-PCR) or mean values ± S.D. (tumor involvement index, Ki67 staining and IHC scores). Statistical analyses done using two-tailed Student’st-test (*P< 0.05, **P< 0.01, ***P< 0.001, ****P< 0.0001) (qRT-PCR) and one-way ANOVA (##P< 0.01). After complete anesthesia, a 20 G angiocatheter was placed into the rat’s urethra. MNU (1.5 mg/kg) (Spectrum) dissolved in 0.9.% sodium chloride was then instilled and the catheter removed, with continued sedation lasting for 60 min to prevent spontaneous micturition and allow absorption. Eighteen weeks after the first MNU instillation, intravesical treatment with PBS or 5 × 10 6 CFU of each BCG strain (0.3 ml via a 20 G angiocatheter) was administered weekly for a total of 6 doses. Animals were monitored regularly and studies were carried out in accordance with the tumor guidelines of JHU Animal Care and Use Committee. Rodents were sacrificed 2 days after the last intravesical treatment, and bladders were harvested within 48 h of the last BCG instillation for mRNA and protein expression analysis as well as histological evaluation. BCG infection of BALB/c mice and CFU enumeration To determine the lung bacillary burden of wild-type and BCG- disA -OE strains 6-week-old female BALB/c mice were exposed using the aerosol route in a Glasscol inhalation exposure system (Glasscol). The inoculum implanted in the lungs at day 1 ( n = 3 mice per group) in female BALB/c mice was determined by plating the whole-lung homogenate on 7H11-selective plates containing carbenicillin (50 mg/ml), Trimethoprim (20 mg/ml), Polymyxin B (25 mg/ml) and Cycloheximide (10 mg/ml). Following infection, mice lungs were harvested ( n = 5 animals/group), homogenized in their entirety in sterile PBS and plated on 7H11-selective plates at different dilutions. The 7H11-selective plates were incubated at 37 °C and single colonies were enumerated at week 3 and 4. Single colonies were expressed at log CFU per organ. SCID Mice time to death study The virulence testing of BCG-WT and BCG- disA -OE strains was done in severely compromised immunodeficient mice aerosol infection model established in our laboratory. The inoculum implanted in the lungs at day 1 ( n = 3 animals per group) was determined by plating the whole-lung homogenate on 7H11-selective plates. For time to death analyses ( n = 10 animals per group) infected animal were monitored until their death. Syngeneic MB49 model of urothelial cancer MB49 tumor cells are urothelial carcinoma line derived from an adult C57BL/6 mouse by exposure of primary bladder epithelial cell explant to 7,12-dimethylbenz[a]anthracene (DMBA) for 24 h followed by a long-term culture. Before implantation, MB49 cells were cultured as monolayers in RPMI 1640 media supplemented with 10% FBS and 1% streptomycin/penicillin at 37 °C with 5% CO 2 . Cells were harvested using Trypsinization and cell viability was determined using Trypan blue dye. Live MB49 cells were resuspended in sterile PBS and adjusted at 1 × 10 5 live cells per 100 μl. Female C57BL/6J mice, age 4–6 weeks (Charles River Laboratories) were subcutaneously injected with 1 × 10 5 MB49 cells in the right flank of hind leg. Tumor growth was monitored every second day to observe the increase the tumor burden at the time of treatment initiation. Once palpable tumor developed (7 to 9 days, average volume ~30 mm 3 1 × 10 6 bacilli of BCG-WT or BCG- disA -OE in a total 50 μl PBS was injected intratumorally. A total of four intratumoral injections of BCG was given every third day. Tumors were measured by electronic caliper, and tumor volume was calculated using the following equation: tumor volume = length x width x height x 0.5326. 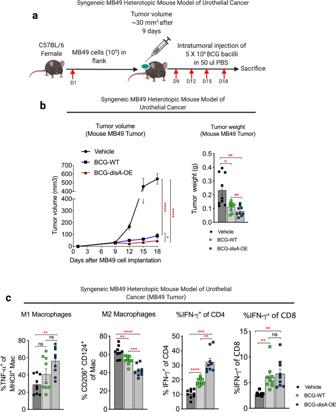Fig. 6: BCG-disA-OE elicits improved antitumor efficacy over BCG-WT in the syngeneic MB49 heterotopic mouse model of urothelial cancer. aSchematic diagram of the syngeneic MB49 mouse model of urothelial cancer.bMB49 tumor volume and tumor weight at time of necropsy (n= 9 animals per group).cTumor-infiltrating M1 and M2 macrophages and CD4 and CD8 T-cell lymphocyte types at necropsy in the MB49 model (n= 9 animals per group). Data are presented as mean values ± S.E.M. Statistical analyses for tumor volume data were done using one-way ANOVA (*P< 0.05, **P< 0.01, ***P< 0.001, ****P< 0.0001). Tumor weight measurement, macrophage, and lymphocyte quantification done using two-tailed Student’st-test (*P< 0.05, **P< 0.01, ***P< 0.001, ****P< 0.0001). 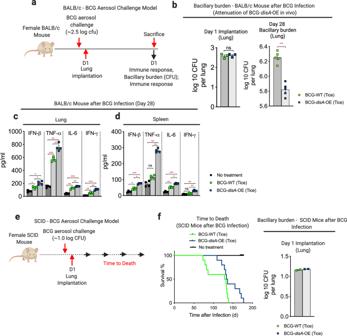Fig. 7: BCG-disA-OE is less pathogenic than BCG-WT in two mouse models and elicits a greater pro-inflammatory cytokine levels in vivo. aSchematic diagram of the immunocompetent BALB/c mouse challenge model.bLung colony forming unit (CFU) counts at day 1 (n= 3 animals/group) and day 28 (n= 5 animals/group). Data are represented as mean values ± S.E.M.cLevels of the pro-inflammatory cytokines IFN-β, TNF-α, IL-6, and IFN-γ in mouse lungs anddspleens determined by ELISA at day 28 (n= 4 animals/group). Data are mean values ± S.E.M.eSchematic diagram of the immunocompromised SCID mouse challenge model.fPercent survival of SCID mice following low-dose challenge (n= 10 animals/group). The day 1 lung CFU counts are shown at right (n= 2 animals/group). All statistical analyses done using two-tailed Student’st-test (*P< 0.05, **P< 0.01, ***P< 0.001, ****P< 0.0001). We did not allow to exceed the maximum allowed tumor volume of ~2 cm in any dimension was based on the guidelines of our Institutional Animal Care and Use Committee for a single implanted tumor that is visible without imaging. Mice were killed at specified time, and tumors and spleens were collected after necropsy for single-cell preparation. Statistics and reproducibility Cell-based assays (cytokine quantifications, gene expression analyses and cellular phenotyping) were performed in a minimum of three ( n = 3) independent biological replicates to derive statistical significance (two-tailed Student’s t-test for two group comparisons). Results are expressed as mean values ± S.EM. Animal studies involving MB49 tumor studies (minimum sample size n = 6 animals per group) was replicated to determine tumor volume (one-way ANOVA for multiple group comparisons), tumor weight and immune infiltrate analyses (two-tailed Student’s t -test) and data are expressed as mean values ± S.EM. MNU rat study involved a minimum sample size of five animals ( n = 5 per group each biological replicate) and were replicated for statistical significance. Treatment outcomes were determined using one-way ANOVA or two-tailed Student’s t -test for different phenotypes as mentioned in figure legends. Data presented as mean ± S.E.M. or S.D. Description of exact number of biological replicates, statistical tests employed, and P -values are given in details. Graphpad Prism (v 9.0) was used for analyses. MNU rats were randomly assigned to different groups and were blinded for treatment arms. The histopathological assessment (IHCs, tumor staging and tumor involvement index) were performed by a genitourinary pathologist blinded for treatment groups. Periodic contamination testing of mammalian cells and BCG strains ensured absence of cross-contamination. None of the data was excluded from the analyses unless the recording quality was poor (e.g., absence of sufficient viable single cells, etc.) or animals developed ulcerate tumors or were moribund. All attempts at replication were successful for in vivo, ex vivo and in vitro assays. The equipment parameters, antibody dilutions, cell numbers and experimental conditions are given in the methods to ensure reproducibility. The results were significant when **** P <  0.0001; *** P <  0.005; ** P <  0.01; * P <  0.05 as given in the figure legends. Reporting summary Additional information on research design is available in the Nature Research Reporting Summary linked to this article.